Splicing the active phases of copper/cobalt-based catalysts achieves high-rate tandem electroreduction of nitrate to ammonia 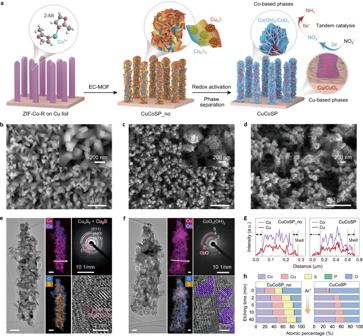Fig. 1: Structural characterizations of catalysts. aSchematic illustration of the preparation of a Cu/Co-based binary ‘tandem catalyst’. SEM images of the ZIF-Co-R precursor (b), CuCoSP_no (c) and CuCoSP (d) on the Cu foil substrate. The inset figures are the SEM images at higher magnification.e,fTypical TEM image, EDX mappings, SAED patterns and HR-TEM image of CuCoSP_no (e) and CuCoSP (f). Unlabelled scale bars are 100 nm. The SAED patterns in (f) show the presence of CuO phases and Co-based oxides/hydroxides (CoOx(OH)y), where 1 = Co(OH)2(100), 2 = Co(OH)2(101), 3 = CuO (20\(\bar{2}\)), 4 = CoOOH (211) and 5 = CoO (220). The purple colours of the HR-TEM image in (f) are marked to guide the eye and correspond to the Co3O4nanocrystals.gEDX line−scan of a selected area marked by the white arrows in (e) and (f).hXPS-determined atomic percentage-depth profile of CuCoSP_no and CuCoSP as a function of Ar+etching time. 2-MI 2-methylimidazole; EC-MOF electrochemically conversion of metal-organic frameworks. Electrocatalytic recycling of waste nitrate (NO 3 − ) to valuable ammonia (NH 3 ) at ambient conditions is a green and appealing alternative to the Haber−Bosch process. However, the reaction requires multi-step electron and proton transfer, making it a grand challenge to drive high-rate NH 3 synthesis in an energy-efficient way. Herein, we present a design concept of tandem catalysts, which involves coupling intermediate phases of different transition metals, existing at low applied overpotentials, as cooperative active sites that enable cascade NO 3 − -to-NH 3 conversion, in turn avoiding the generally encountered scaling relations. We implement the concept by electrochemical transformation of Cu−Co binary sulfides into potential-dependent core−shell Cu/CuO x and Co/CoO phases. Electrochemical evaluation, kinetic studies, and in−situ Raman spectra reveal that the inner Cu/CuO x phases preferentially catalyze NO 3 − reduction to NO 2 − , which is rapidly reduced to NH 3 at the nearby Co/CoO shell. This unique tandem catalyst system leads to a NO 3 − -to-NH 3 Faradaic efficiency of 93.3 ± 2.1% in a wide range of NO 3 − concentrations at pH 13, a high NH 3 yield rate of 1.17 mmol cm −2 h −1 in 0.1 M NO 3 − at −0.175 V vs. RHE, and a half-cell energy efficiency of ~36%, surpassing most previous reports. Ammonia (NH 3 ) is the critical feedstocks of artificial fertilizers and various chemicals and one of the most promising carbon-free energy carriers [1] , [2] , [3] . Currently, industrial NH 3 synthesis heavily relies on the energy and carbon−emission intensive Haber−Bosch (H–B) process [4] , [5] , [6] , [7] . Alternatively, electrocatalytic N 2 -to-NH 3 conversion ( e N 2 –NH 3 ), using water (H 2 O) as a proton source, has recently attracted significant research interests owing to its mild conditions and high compatibility with renewable electricity [6] , [8] , [9] , [10] , [11] , [12] , [13] , [14] , [15] . However, the inherent characters of N 2 , including high dissociation energy of the N≡N bond (945 kJ mol −1 ) and low water solubility, make the e N 2 –NH 3 work at an insufficient selectivity and two orders of magnitude lower yield rate than that of H–B process [9] , [10] , [11] , [16] . To bridge the gap, the knowledge of the nitrogen cycle brings a renewed attention to the recycling of reactive N–containing species (e.g., NO and nitrate) to NH 3 [17] , [18] , [19] , [20] . Among them, the nitrate (NO 3 − ) anion is particularly attractive because it exhibits comparatively low dissociation energy of the N=O bond (204 kJ mol −1 ) and is widely abundant as pollution in agricultural and industrial wastewaters [20] , [21] , [22] , [23] , [24] , [25] , [26] . Furthermore, initial developments of plasma techniques promise to convert air to NO 3 − with low energy consumption [27] , [28] . Therefore, using NO 3 − as the precursor endows NH 3 electrosynthesis with sustainable features and opens up an economical route to remedy environmental pollution. NO 3 − -to-NH 3 conversion in microorganisms is a tandem process; i.e., NO 3 − reduction to NO 2 − using nitrate reductase and subsequent NO 2 − -to-NH 3 conversion employing nitrite reductase or nitrogenase, independently [29] , [30] , [31] . This enzyme-based tandem system allows efficient NH 3 generation at ambient conditions in nature owing to its specific coordination binding with NO 3 − and NO 2 − , respectively [29] , [31] , [32] . However, NO 3 − typically shows low binding affinity to transition metals in aqueous electrolytes due to its symmetrical (D 3h ) resonant structure and strong hydrogen bonding to H 2 O [31] , [33] , [34] . Moreover, the NO 3 − -to-NH 3 pathway involves a complex eight−electrons transfer and multiple intermediates [17] , [35] , [36] . As a result, there is a scaling relation between the binding strengths of NO 3 − , NO 2 − and other oxygen−containing intermediates (e.g., NO) on the transition metal surface [37] . Optimizing the adsorption of one species will typically take the others away from their optima [38] , [39] , making the simultaneous acceleration of sequential NO 3 − -to-NO 2 − and NO 2 − -to-NH 3 reactions considerably challenging. Copper (Cu)-based catalysts have been intensively investigated for the NO 3 − reduction reaction (NO 3 RR) due to its favorable ability to bind NO 3 − and catalyze NO 3 − -to-NO 2 − conversion [40] , [41] , [42] , [43] . However, pure Cu catalysts commonly suffer from rapid deactivation because of their strong adsorption of the NO 3 RR intermediates (e.g., NO 2 − and NO) [42] , [43] , [44] . Substantial efforts have recently been made to alleviate these limitations by regulating the proton- and/or electron-transfer, as well as the binding strengths of partially reduced intermediates adsorbed on Cu centres. This was performed either by alloying Cu with noble or other transition metals (e.g., Pt, Pd and Ni) [40] , [45] , [46] , [47] , [48] , [49] or through the formation of hybrids with molecular solids or metal oxides (e.g., Cu 2 O) [44] , [50] , [51] . These strategies have increased the Faradaic efficiency (FE) of NH 3 to an impressive 70–100% and the NH 3 yield rate (Y NH3 ) to a level of 30–200 μmol cm −2 h −1 [44] , [45] , [51] . However, restricted by the scaling relations, these advances require highly concentrated NO 3 − (e.g., 1 M) and/or relatively high overpotentials (<−0.4 V vs. RHE) to balance the rates of NO 3 − -to-NO 2 − and NO 2 − -to-NH 3 reactions, resulting in an increased energy consumption [44] , [45] , [51] . To compete with the H–B process, further progress on Y NH3 (>1 mmol cm −2 h −1 ) [52] and on decreasing energy consumption are highly desirable. Energy-efficient NO 3 RR points to low operating overpotentials (e.g., >−0.2 V vs. RHE), at which transition metal (e.g., Cu and Co)-based catalysts often suffer from potential−dependent phase evolution, leading to the coexistence of multiple phases, such as metallic, oxide and hydroxide phases [53] , [54] , [55] , [56] . In situ monitoring of the phase evolution of transition metals during the NO 3 RR, while correlating these intermediate phases with specific catalytic steps [53] , [54] , [57] , [58] , may not only guide the rational design of selective catalysts for NH 3 but also provide insight into the NO 3 RR. Inspired by the tandem NO 3 − -to-NH 3 conversion in nature [29] , we sought, therefore, to circumvent the scaling relations by combining two or more cooperative intermediate phases exhibiting complementary catalytic selectivity into one tandem system, intending to achieve NH 3 synthesis at low overpotentials. Importantly, it has been clearly demonstrated that the reaction rate and selectivity of a tandem catalyst system, linked to the transport of key intermediates, could be optimized by judiciously tuning the proximity, hierarchy and content ratio of multiple active phases [39] , [59] , [60] , [61] , [62] . Accordingly, the Y NH3 could be further improved, however, to the best of our knowledge, tandem catalysts based on earth−abundant elements have never been reported for electrocatalytic consecutive NO 3 – -to-NH 3 conversion. In this work, we introduce a facile electrochemically driven phase-separation strategy for a tandem catalyst design, which, different from previous approaches based on sequential assembling or deposition [60] , [61] , enables the in situ formation of multiple active intermediate phases and rich phase interfaces for rapid spillover and transport of reaction intermediates. As a proof-of-concept, we implemented this catalyst synthesis strategy by the electrochemical transformation of pre−synthesized Cu–Co binary metal sulfides into core–shell Cu/CuO x and Co/CoO phases on Cu foil. The employment of Co-based phases as a sub−component of the tandem catalysts was inspired by the previously reported high selectivity of Co-based materials and complexes for NH 3 generation during the NO 3 RR and the specific NO 2 − -to-NH 3 conversion [63] , [64] . Our electrocatalytic tests, kinetic studies, in situ scanning electrochemical microscopy (SECM) and in situ Raman spectra reveal that at low overpotentials, the inner Cu/CuO x phases preferentially catalyze NO 3 − reduction to NO 2 − , while the outer-layer Co/CoO phases selectively catalyze NO 2 − reduction to NH 3 , both of which can be combined for rapid “working-in-tandem” NH 3 synthesis. As a result, we report NO 3 − -to-NH 3 conversion with a FE of 93.3 ± 2.1% in a wide range of NO 3 − concentrations at −0.175 V vs. RHE, a high NH 3 yield rate of 1.17 mmol cm −2 h −1 in 0.1 M NO 3 − at pH 13 and a half−cell energy efficiency of ~36%, which surpass most prevreports. Catalyst design and characterization The synthesis of Cu/Co-based tandem catalysts is schematically illustrated in Fig. 1a . A nanorod array of metal-organic frameworks (MOFs) was first grown on Cu foil by optimizing the molar ratio of 2-methylimidazole and Co 2+ to 20: 1 (hereafter named as ZIF-Co-R/Cu; Fig. 1b and Supplementary Fig. S1 ). The ZIF-Co-R/Cu was converted into Cu–Co binary metal sulfides following a previously reported electrochemically conversion of MOF (EC-MOF) strategy [65] , [66] , [67] . Upon adding 0.05 M Na 2 HPO 4 as structure-tuning agents, the nanorod contour of ZIF–Co−R could be retained during the EC-MOF (Fig. 1c ), which was otherwise changed into super-thin nanosheets (Supplementary Fig. S2 ). We denoted the PO 4 3− -modified Cu–Co binary metal sulfides as CuCoSP_no and their products after further electrochemical redox activation as CuCoSP. This unique nanorod array configuration of CuCoSP can provide a more efficient pathway for mass and charge transport during the NO 3 RR, contributing to the best performance of CuCoSP for NO 3 RR as discussed below. Fig. 1: Structural characterizations of catalysts. a Schematic illustration of the preparation of a Cu/Co-based binary ‘tandem catalyst’. SEM images of the ZIF-Co-R precursor ( b ), CuCoSP_no ( c ) and CuCoSP ( d ) on the Cu foil substrate. The inset figures are the SEM images at higher magnification. e , f Typical TEM image, EDX mappings, SAED patterns and HR-TEM image of CuCoSP_no ( e ) and CuCoSP ( f ). Unlabelled scale bars are 100 nm. The SAED patterns in ( f ) show the presence of CuO phases and Co-based oxides/hydroxides (CoO x (OH) y ), where 1 = Co(OH) 2 (100), 2 = Co(OH) 2 (101), 3 = CuO (20 \(\bar{2}\) ), 4 = CoOOH (211) and 5 = CoO (220). The purple colours of the HR-TEM image in ( f ) are marked to guide the eye and correspond to the Co 3 O 4 nanocrystals. g EDX line−scan of a selected area marked by the white arrows in ( e ) and ( f ). h XPS-determined atomic percentage-depth profile of CuCoSP_no and CuCoSP as a function of Ar + etching time. 2-MI 2-methylimidazole; EC-MOF electrochemically conversion of metal-organic frameworks. Full size image Low-resolution transmission electron microscopy (TEM) and high-resolution scanning electron microscopy (HR-SEM) images reveal that a curly nanosheet-assembled shell wraps the nanorod skeleton of CuCoSP_no (Fig. 1c, e and Supplementary Fig. S3a ). The corresponding EDX mapping shows strong Co, Cu and S signals well-distributed in the whole nanorod and a weak signal of O due to surface oxidation. Remarkably, Cu is also spread over the nanorod, indicating that the Cu comprised in CuCoSP_no is from the dissolution of Cu foil followed by redeposition and inward diffusion of the released Cu ions during the EC-MOF. The enrichment of Cu on the CuCoSP_no surface is supported by the EDX-linear scan (Fig. 1g and Supplementary Fig. S3 ). Moreover, HR-TEM images, coupled with selected area electron diffraction (SAED), reveal that the curly nanosheets and skeleton of CuCoSP_no are mainly composed of ~3–5 nm Co 9 S 8 and Cu 2 S nanocrystals, which are not detectable by X-ray diffraction (XRD) (Supplementary Fig. S4d ) [59] , [66] . After the electrochemical activation, the obtained CuCoSP preserves the contour of CuCoSP_no, except for the in situ formation of a hexagon-shaped nanosheet-assembled shell (Fig. 1d, f and Supplementary Fig. S5a ). Compared to CuCoSP_no, the CuCoSP possesses more complex SAED patterns corresponding to multiple mixed phases (Fig. 1f ), which include Co(OH) 2 , CoOOH, CoO and CuO EDX mappings and linear EDX scans (Fig. 1f and Supplementary Fig. S5f ) show weaker S and enhanced O signals. These results suggest a significant transformation of Cu–Co binary sulfides into oxides and hydroxides, as corroborated by the XRD patterns (Supplementary Fig. S4e ), as well as Raman and X-ray photoelectron spectroscopy (XPS). An HR-TEM image of a hexagon-shaped nanosheet on CuCoSP shows a typical (101) facet of Co(OH) 2 and some Co 3 O 4 nanocrystals at the edge. The EDX mapping of CuCoSP shows an intertwined distribution of Cu and Co on the nanorod (Fig. 1f ), and the linear EDX scan reveals a higher content of Co in the shell region (Fig. 1g ). Therefore, the shell assembled by xagon-shaped nanosheets is a Co element-rich phase, and the redox activation might induce the redistribution of Co-based and Cu-based phases. To investigate the spatial arrangement of Cu-based and Co-based phases, we carried out XPS depth profiling. We calculated the atomic percentages of Cu, Co, O, S and P in both CuCoSP_no and CuCoSP as a function of Ar + etching time (Fig. 1h and Supplementary Fig. S6 ). We found that the CuCoSP_no has a Cu-rich surface (Co: Cu = 0.862: 1) and Co-rich core (Co: Cu = 1.83: 1 at 40 min etching time), which is in line with the EDX-linear scan results. The surface of CuCoSP is enriched with Co with a Co/Cu ratio of 5.23: 1. After 5 min etching time, the Co/Cu ratio decreases to 3.07: 1 and slightly decreases in the following 35 min of Ar + etching. The results reveal an electrochemical redox activation-induced outward diffusion of Co ions and a relative inward diffusion of Cu ions, contributing to the phase separation in CuCoSP. The outward diffusion of Co ions is attributed to the easier oxidation of cobalt sulfides than copper sulfides into corresponding oxides or hydroxides. EDX mapping images of CuCoSP_no after one-cycle redox activation provide further evidence (Supplementary Fig. S7 ), with the maps of Co and O overlapping on the outer-shell layer and those of Cu and residual S in the inner-core layer. This controllable phase separation in metal sulfide matrix driven by electrochemically redox activation may offer a strategy for a tandem catalyst design, which enables in situ formation of multiple active phases and rich phase interfaces for rapid spillover and transfer of reaction intermediates. This core–shell arrangement of the Cu-based phases and Co-based phases, together with the rich phase interface between them, is the key to achieve a near-unity selectivity for subsequent NO 3 − -to-NH 3 catalysis on CuCoSP. The Cu foil substrate of CuCoSP may play a similar role to the Cu-based phases (Fig. 1a ). As a control, we used a Cu foil or ZIF-Co-R grown on carbon paper (CC) as precursors and treated them by the same EC-MOF and activation procedures (Supplementary Fig. S8 ). The related materials were denoted as CuSP and CoSP, respectively. NO 3 RR performance Linear sweep voltammetry (LSV) and one-hour electrolysis were performed for assessing the activity and selectivity of the as-synthesized catalysts in 0.01 M KNO 3 and 0.1 M KOH (pH 13) (Fig. 2a–c ). Unless otherwise noted, all potentials are corrected vs the reversible hydrogen electrode (RHE). Performing NO 3 RR in alkaline media was chosen due to the reported lower probability of the formation of toxic intermediates in solution (e.g., nitrogen oxides and NH 2 OH), as compared to those in acidic or neutral media, as well as the need of removing NO 3 − ions in alkaline nuclear wastewater [21] , [42] . We set the concentration of nitrate to be 0.01 M, which ensures the concentration of formed NH 3 to be easily higher than that of environmental contaminants which in turn helps to compare the intrinsic activity of the catalysts via bypassing the positive effects of high-concentration NO 3 − (e.g., 1 M) with respect to facilitating the NO 3 RR [52] , [68] . Fig. 2: NO 3 − -to-NH 3 conversion performance. LSVs at a scan rate of 5 mV s −1 ( a ), Faradaic efficiencies (FE) for NH 3 ( b ) and NO 2 − ( c ) on CuSP, CoSP and CuCoSP in 0.01 M NO 3 − and 0.1 M KOH (pH 13) at various applied potentials. d A comparison of half-cell energy efficiencies of NH 3 (EE NH3 ) and partial current densities of NH 3 ( j NH3 ) on CuSP, CoSP and CuCoSP catalysts at various potentials. e The FE of NO 2 − and NH 3 , the NH 3 yield rate (Y NH3 ), as well as the ratio of the formed NH 3 concentration [NH 3 ] to the converted NO 3 − concentration [NO 3 − ] on the CuCoSP catalyst at −0.175 V vs. RHE at [NO 3 − ] in the range of 1−100 mM at pH 13. f The ECSA-normalized Y NH3 on CuSP, CoSP, CuCoSP and metallic CuCo hybrids in 0.01 M NO 3 − and 0.1 M KOH at various potentials. Error bars denote the standard deviations calculated from three independent measurements. Full size image The LSV of CuSP in the presence of NO 3 − is similar to that of the NO 3 RR on the Cu (100) facet [42] , where a diffusion-limited maximum total current density ( j total ) of −55.3 mA/cm −2 is reached at around −0.3 V. At <−0.3 V, the surface of CuSP becomes blocked by the strongly adsorbed intermediates of the H 2 evolution reaction (HER) and/or NO 3 RR until the surface is renewed because of the drastic HER at <−0.6 V [42] . CoSP requires a ~150 mV more negative potential to drive the NO 3 RR, but it shows a sharply increased j total for the HER at <−0.2 V, where metallic Co is supposedly formed (Supplementary Fig. S9 ). The CuCoSP has the catalytic features of both CuSP and CoSP, showing the highest NO 3 RR activity between −0.16 V and 0.085 V. Moreover, the Tafel slope of CuCoSP for the HER in 0.1 M KOH is 69 mV dec −1 , and smaller than those of CuSP (125 mV dec −1 ) and CoSP (104 mV dec −1 ), suggesting faster kinetics for the HER (Supplementary Fig. S9 ). Thus, there is a strong synergy between the Cu-based and Co-based phases in CuCoSP for NO 3 RR at >−0.2 V and HER at <−0.2 V. Determination of the product selectivity for CuSP, CoSP and CuCoSP shows a significant difference in the FE for NH 3 and NO 2 − (Fig. 2b, c and Supplementary Figs. S10 – 13 ). At low over−potentials (>−0.2 V), CuSP exclusively catalyzes the formation of NO 2 − , while CoSP shows a high inherent NH 3 selectivity without any interference from the underlying CC (Supplementary Fig. S14d ). The CuCoSP inherits the advantages of CoSP and reaches a maximum FE of 95.9% for NH 3 at −0.075 V, 14.5% higher than that of CoSP. This finding further suggests the synergy of the Cu-based and Co-based phases in CuCoSP for selective NO 3 − -to-NH 3 conversion. Moreover, the CuCoSP shows a FE of 88.7% for NH 3 and an NH 3 partial current densities ( j NH3 ) of −9.54 mA cm −2 at −0.025 V, a potential at which CuSP exhibits exclusive NO 2 − generation and CoSP shows a negligible NO 3 RR activity (Fig. 2a–d and Supplementary Figs. S11 – 13 ). CuCoSP retains this advantage even at 0.025 V (a FE of 66.4% for NH 3 and a j NH3 of −3.84 mA cm −2 ). Similar to CuSP, the Cu foil and inner Cu-based phases of CuCoSP can catalyze the preferential formation of NO 2 − , which might then be further reduced to NH 3 at the outer Co-based phases. This hypothesis, as further demonstrated below, may well account for the ~2-fold higher j NH3 for CuCoSP than that of CoSP at >−0.175 V (Fig. 2d ). At higher overpotentials (<−0.2 V), CuCoSP and CoSP show a sharp decline of the FE for NH 3 but minor changes in their FE for NO 2 − (<1%) (Fig. 2b–d ), indicating that the NO 3 RR on CuCoSP and CoSP is challenged by the drastically enhanced HER (Supplementary Fig. S9 ). The competing HER was previously suppressed by increasing the NO 3 − concentrations and/or the pH value of electrolytes [45] , [52] . As anticipated, j total of CuCoSP linearly increases with the NO 3 − concentrations (Supplementary Fig. S15 ), indicative of a first-order reaction kinetics. At −0.175 V, the CuCoSP catalyst reaches a nearly equal FE of 93.3 ± 2.1% for NH 3 and a linearly increased NH 3 yield rate (Y NH3 ) with a value of 15.7, 33.4, 74.1, 155 and 327 μmol h −1 cm −2 in 1, 2, 5, 10 and 20 mM NO 3 − , respectively (Fig. 2e ). When the NO 3 − concentration increases to 50 and 100 mM, the Y NH3 of CuCoSP reaches 0.690 and 1.17 mmol h −1 cm −2 , respectively. The latter is comparable to the highest reported value of 1.17 mmol h −1 cm −2 on strained Ru nanoclusters evaluated at −0.2 V in 1 M NO 3 − and 1 M KOH (pH 14) [52] . The turnover numbers (TON) of nitrate on CuCoSP, defined by the ratio of the yielded NH 3 concentration [NH 3 ] to the converted NO 3 − concentration [NO 3 − ], are close to 1 at [NO 3 − ] < 20 mM. This indicates that the formed NH 3 is mainly derived from the NO 3 − electroreduction rather than any environmental contaminations (Fig. 2e and Supplementary Fig. S15d ). However, the TON value decreases to ~0.8 in 100 mM nitrate electrolytes, suggesting that high [NO 3 − ] might induce the formation of gaseous by-products (e.g., N 2 and NO x ) [36] . Finally, the CuCoSP achieves a half-cell energy efficiency of NH 3 (EE NH3 ) close to 40%. These results endow the proposed CuCoSP ranking among the best NH 3 synthesizing electrocatalysts (Supplementary Table S 1 ). To assess the origin of the detected NH 3 and correct the Y NH3 , we employed 1 H NMR to detect the NH 3 generation on CuCoSP in 0.1 M KOH containing 0.01 M 15 N-labelled 15 NO 3 − or 14 NO 3 − (Supplementary Fig. S16 ). The 14 NH 3 yield quantified by 1 H NMR is very close to that determined by colorimetric methods [69] , confirming the reliability of our results. The negligible NH 3 generation in blank 0.1 M KOH and the typical 1 H NMR double peaks of 15 NH 4 + after the electrolysis of 15 NO 3 − suggest that the obtained NH 3 indeed originates from the NO 3 RR [25] , [28] , [44] . To derive the intrinsic activities of the catalysts, we normalize their Y NH3 by the electrochemical active surface area (ECSA) (correlated with the double-layer capacity (C dl )) (Fig. 2f and Supplementary Fig. S17 ). At low overpotentials, the Y NH3 of CuCoSP can be ~45 times and two orders of magnitude higher than those of CoSP and CuSP, respectively, confirming the high intrinsic performance of CuCoSP. Remarkably, CuSP lost activity rapidly at >−0.525 V during the NO 3 − electrolysis (Supplementary Fig. S11 ), which occurred neither at CoSP nor at CuCoSP (Supplementary Fig. S12 and S13 ). This finding indicates that the Co-based phases existing in CoSP and CuCoSP may help to avoid similar poisoning effects. When the NO 3 RR was performed at −0.175 V for 10 h over the CuCoSP catalyst, no appreciable decay in activity and selectivity for NO 3 − -to-NH 3 conversion was observed, and the structural features of CuCoSP were retained (Supplementary Fig. S18 ). Understanding the high-rate NH 3 generation on CuCoSP Electrocatalytic NO 3 RR follows a consecutive pathway (Fig. 3a ), where NO 2 − is generated as a stable intermediate [17] , [36] . A fast NO 3 − -to-NH 3 conversion requires the simultaneous acceleration of the sequential NO 3 − -to-NO 2 − and NO 2 − -to-NH 3 reactions [35] , [36] . To rationalize the high Y NH3 on CuCoSP at low overpotentials, we firstly compared the potentials of the three catalysts required to reach −1 mA cm −2 (kinetic area with negligible mass transport limitation) in 0.01 M NO 3 − and NO 2 − , respectively (Supplementary Fig. S20 ). CuSP shows a 176 mV more positive potential than CoSP for NO 3 − reduction, while CoSP has a 251 mV more positive potential than CuSP for NO 2 − reduction. Therefore, CuSP and CoSP may play a complementary role for the consecutive NO 3 RR. Significantly, CuCoSP combines the positive properties of CuSP and CoSP for NO 3 − and NO 2 − reduction, respectively, implying that there are likely two types of active phases in CuCoSP: Cu-based phases which are similar to those in CuSP, and Co-based phases which are similar to those in CoSP. The two types of active phases in CuCoSP synergistically catalyze the tandem NO 3 RR. Fig. 3: Evaluation of the reaction kinetics and mechanisms of the catalysis of the NO 3 RR. a The LSV-derived potentials at a current density of −1 mA cm −2 and the calculated reaction constants (k, k 1 for NO 3 − -to-NO 2 − and k 2 for NO 2 − -to-NO conversion) for NO 3 − and NO 2 − reduction on CuSP, CoSP and CuCoSP catalysts. k was calculated based on the concentration evolution of NO 3 − or NO 2 − ions as a function of electrolysis time at −0.175 V vs. RHE in 0.01 M NO 3 − and NO 2 − at pH 13. Error bars denote the standard deviations of k calculated at different time points during 1 h electrolysis. b A comparison of the FE and the Y NH3 on the control catalysts: CuCoSP_0.5, CuCoSP_4, CuCoSP_no, CuCoS and metallic CuCo hybrids. The LSV-derived Tafel slopes of CuSP, CoSP and CuCoSP in 0.01 M nitrate ( c ) and nitrite ( d ) at pH 13, respectively. The LSVs were recorded at a scan rate of 1 mV s −1 . e Schematic representation of the SECM setup that is operated in a sample generation-tip collection (SG-TC) mode using a Pt-UME (WE 2) to detect NO 2 − and NH 3 produced during NO 3 RR on Cu_Co(OH) 2 model catalyst (WE 1). Inset: SEM image of Pt-UME tip; scale bar is 500 nm. f , g Current maps of NH 3 oxidation ( f ) and NO 2 − reduction ( g ) recorded at 0.76 V and 0.06 V (vs. RHE) at the Pt-UME, respectively, when a potential of −0.12 V (vs. RHE) is applied to the Cu_Co(OH) 2 model catalyst in 50 mM NO 3 − at pH 13. Full size image To validate this hypothesis, we further evaluated the rate constants k 1 and k 2 of each catalyst for NO 3 − -to-NO 2 − and NO 2 − -to-NH 3 conversion, respectively (Supplementary Fig. S21 and Table S2 ). We found that the rate constants of the three catalysts follow a similar trend as their potentials at −1 mA cm −2 ; a larger rate constant corresponding to a more positive potential for reaching −1 mA cm −2 (Fig. 3a ). The largest k 1 but the smallest k 2 values of CuSP correspond to a fast reduction of NO 3 − to NO 2 − and subsequent desorption of NO 2 − to the electrolyte, resulting in the observed high FE of NO 2 − (Fig. 2c and Supplementary Fig. S11 ). On the CuCoSP surface, NO 2 − intermediates are preferentially formed on Cu-based phases and then spilt over to nearby Co-based phases. Compared to the k 2 /k 1 ratio of CuSP (0.468), the larger k 2 /k 1 ratios of CoSP (3.14) and CuCoSP (1.78) suggest a fast reduction of the intermediate NO 2 − to NH 3 over their Co-based phases, thus well explaining their near-unity selectivity for NH 3 generation. We used the k 1 values of CoSP and CuCoSP to estimate their local surface NO 2 − concentration during the NO 3 RR and find a 1.54-fold higher value on CuCoSP than on CoSP (Supplementary Table S2 ), which is consistent with the observed 1.66-fold larger j NH3 of CuCoSP compared to CoSP at −0.175 V (Fig. 2d ). This finding unveils the crucial role of Cu-based phases in CuCoSP for creating a high local NO 2 − concentration, which accelerates subsequent NH 3 generation on its Co-based phases, ultimately contributing to the tandem catalysis of NO 3 RR. Considering the lowest k 1 value of CoSP, the smaller k 1 value of CuCoSP than CuSP can be rationalized since the less active Co-based phases of CuCoSP may block its active Cu-based phases (especially the Cu foil substrate) for NO 3 − reduction. As such, we synthesized the CuCoSP_0.5 and CuCoSP_4 with 0.5 h and 4 h growth of ZIF-Co-R on Cu foil, respectively. The CuCoSP_0.5 shows catalytic features close to CuSP, thus giving a higher FE for NO 2 − than CuCoSP (Fig. 3b and Supplementary Fig. S22 ). This finding indicates that possible Co doping in Cu-based phases of CuCoSP_0.5 does not change their catalytic nature. Likewise, the CuCoSP _4 shows a similar catalytic feature to CoSP with a low sum FE for NO 3 RR. Therefore, the content ratio of Cu-based and Co-based phases in CuCoSP, rather than the Cu or Co doping, determines the rates of the NO 3 − -to-NO 2 − and NO 2 − -to-NH 3 reactions. This is a typical feature of tandem catalysts [39] , [59] . Electrokinetic analysis was conducted to determine the rate-determining step (RDS) of the NO 3 − and NO 2 − reduction catalyzed by the three catalysts. In 0.01 M NO 3 − (Fig. 3c ), CuSP and CuCoSP show Tafel slopes of 94 and 112 mV dec −1 , respectively, a little lower than 120 mV dec −1 , suggesting that the RDS is the first one-electron transfer occurring during the NO 3 − -to-NO 2 − conversion [34] , [48] , [70] . The much higher Tafel slope of CoSP (167 mV dec −1 ) indicates that the NO 3 RR over CoSP is limited by the initial adsorption and activation of NO 3 − [48] . In 0.01 M NO 2 − (Fig. 3d ), CoSP and CuCoSP show Tafel slopes of 106 and 101 mV dec −1 , respectively, suggesting that the RDS is the first one-electron transfer for the reduction of NO 2 − to NO [34] , [48] . CuSP has a Tafel slope of 72 mV dec −1 , close to the critical value of 60 mV dec −1 , implying that the RDS is a chemical step [71] , [72] . Based on the theoretical NO 3 RR pathways on Cu [44] , this RDS is likely the coupling of strongly adsorbed *NO and *H. Remarkably, the smaller Tafel slope of CuSP than those of CoSP and CuCoSP points to a faster NO 2 − reduction kinetics on CuSP, but CuSP suffers from a faster deactivation in 0.01 M NO 2 − than in 0.01 M NO 3 − (Supplementary Fig. S21 ), thus giving the smallest apparent k 2 value. Accordingly, the observed poisoning of CuSP might be ascribed to the strongly adsorbed *NO species. Therefore, CuCoSP combines the nature of CuSP for NO 3 − reduction with that of CoSP for NO 2 − reduction. 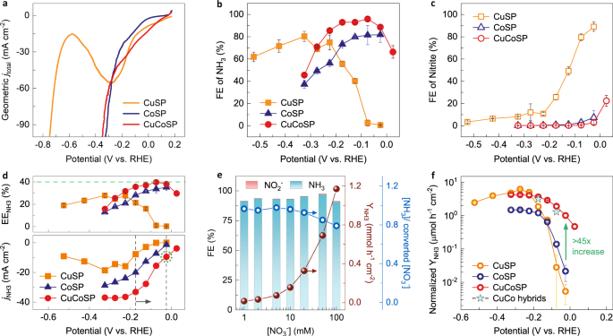Fig. 2: NO3−-to-NH3conversion performance. LSVs at a scan rate of 5 mV s−1(a), Faradaic efficiencies (FE) for NH3(b) and NO2−(c) on CuSP, CoSP and CuCoSP in 0.01 M NO3−and 0.1 M KOH (pH 13) at various applied potentials.dA comparison of half-cell energy efficiencies of NH3(EENH3) and partial current densities of NH3(jNH3) on CuSP, CoSP and CuCoSP catalysts at various potentials.eThe FE of NO2−and NH3, the NH3yield rate (YNH3), as well as the ratio of the formed NH3concentration [NH3] to the converted NO3−concentration [NO3−] on the CuCoSP catalyst at −0.175 V vs. RHE at [NO3−] in the range of 1−100 mM at pH 13.fThe ECSA-normalized YNH3on CuSP, CoSP, CuCoSP and metallic CuCo hybrids in 0.01 M NO3−and 0.1 M KOH at various potentials. Error bars denote the standard deviations calculated from three independent measurements. To assess the possible roles of anionic ligands (PO 4 3− and S 2− ) in our system, we tested the NO 3 RR performance of CuCoSP_no catalysts with the maximum PO 4 3− and S 2− ligands and CuCoS catalysts with only S 2− ligand. The lower FE (for NH 3 ) and Y NH3 of CuCoSP_no compared with those of CuCoSP (Fig. 3b ), in combination with the near-unity NH 3 selectivity but low Y NH3 of CuCoS (Fig. 3b and Supplementary Fig. S23 ), suggest that PO 4 3− and S 2− ligands most likely do not play a prominent role. We evaluated the final morphology of CuCoSP after repeating three electrolysis of one hour at −0.325 V and observed a separation of Cu-based phases (nanorods) and Co-based phases (hexagonal nanosheets) based on EDX mapping and HR-TEM images (Supplementary Fig. S24 ). This result rules out the formation of a bulk CuCo alloy, as corroborated by the XRD patterns (Supplementary Fig. 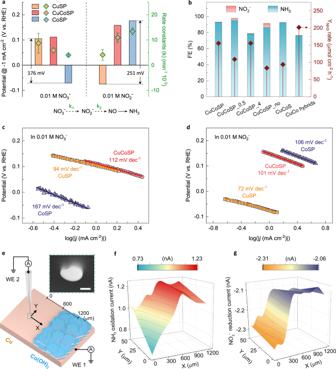Fig. 3: Evaluation of the reaction kinetics and mechanisms of the catalysis of the NO3RR. aThe LSV-derived potentials at a current density of −1 mA cm−2and the calculated reaction constants (k, k1for NO3−-to-NO2−and k2for NO2−-to-NO conversion) for NO3−and NO2−reduction on CuSP, CoSP and CuCoSP catalysts. k was calculated based on the concentration evolution of NO3−or NO2−ions as a function of electrolysis time at −0.175 V vs. RHE in 0.01 M NO3−and NO2−at pH 13. Error bars denote the standard deviations of k calculated at different time points during 1 h electrolysis.bA comparison of the FE and the YNH3on the control catalysts: CuCoSP_0.5, CuCoSP_4, CuCoSP_no, CuCoS and metallic CuCo hybrids. The LSV-derived Tafel slopes of CuSP, CoSP and CuCoSP in 0.01 M nitrate (c) and nitrite (d) at pH 13, respectively. The LSVs were recorded at a scan rate of 1 mV s−1.eSchematic representation of the SECM setup that is operated in a sample generation-tip collection (SG-TC) mode using a Pt-UME (WE 2) to detect NO2−and NH3produced during NO3RR on Cu_Co(OH)2model catalyst (WE 1). Inset: SEM image of Pt-UME tip; scale bar is 500 nm.f,gCurrent maps of NH3oxidation (f) and NO2−reduction (g) recorded at 0.76 V and 0.06 V (vs. RHE) at the Pt-UME, respectively, when a potential of −0.12 V (vs. RHE) is applied to the Cu_Co(OH)2model catalyst in 50 mM NO3−at pH 13. S4f ). To identify the impact of surface CuCo metallizing and/or alloying possibly during the NO 3 RR, we electrodeposited a hybrid of Cu–Co metals and alloy (Co: Cu = 2.82: 1, close to that on CuCoSP surface) on CC (Supplementary Fig. S25 ). The metallic CuCo hybrids show Tafel slopes of 61 mV dec −1 in 0.01 M NO 3 − and 79 mV dec −1 in 0.01 M NO 2 − , indicating a significantly different catalytic mechanism and kinetics than CuCoSP. Despite its higher apparent Y NH3 , the CuCo hybrids have a lower FE for NH 3 and ECSA-normalized Y NH3 than CuCoSP (Fig. 2f and 3b). The ECSA-normalized Y NH3 of CuCo hybrids is about 85 and 67% of that formed on CuCoSP at −0.175 V and −0.025 V, respectively. As such, the excellent intrinsic performance of CuCoSP towards NH 3 generation, especially at low overpotentials, is unlikely from surface Cu–Co metallizing or alloying. It can be concluded that the high-rate NO 3 − -to-NH 3 conversion on CuCoSP is due to the coexistence of the complementary Cu-based and Co-based phases: the former catalyzes NO 3 − -to-NO 2 − reduction and the latter catalyzes the NO 2 − -to-NH 3 conversion, contributing to the tandem catalysis of NO 3 RR. To offer a direct evidence for this tandem catalysis of NO 3 RR, we performed SECM experiments in a surface-generation tip-collection mode, which involves using a positioned Pt ultramicroelectrode (Pt-UME) to detect the NO 2 − and NH 3 formed on the surface of a Cu_Co(OH) 2 model catalyst (Fig. 3e ) during the NO 3 − electrolysis. This Cu_Co(OH) 2 model catalyst has two adjacent layers to simulate the CuSP (Cu layer) and CoSP (Co(OH) 2 layer) catalysts, while the border between the two layers may play a similar role of as the adjacent phases in CuCoSP (Supplementary Fig. S26 ). During the SECM measurements, the catalyst layer was polarized to −0.12 V (vs. RHE), while at the positioned Pt-UME cyclic voltammetry (CV) in the potential range between −0.12 V and 1.58 V (vs. RHE) at a rate of 200 mV s −1 was performed. We were applying −0.12 V at catalysts as we found that at this potential, CuSP and CoSP is relatively more stable and active compared to potentials of −0.075 V and −0.025 V, which is beneficial for in situ detection of the intermediately formed NO 2 − and NH 3 . The same reason is the use of a concentration of 50 mM NO 3 − . At −0.12 V, CuSP mainly produces NO 2 − , and CoSP exhibits a much lower NO 3 RR activity compared to CuCoSP, as indicated in Fig. 2a–c and Supplementary Fig. S11 – 13 . 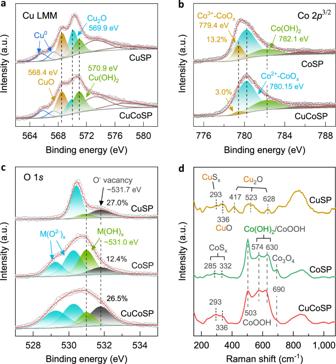Fig. 4: Surface phase compositions of CuSP, CoSP and CuCoSP catalysts. Cu LMM (a), Co 2p3/2(b) and O 1s(c) XPS spectra.dEx situ Raman spectra. We firstly performed cyclic voltammograms at the Pt-UME separately in 10 mM NO 3 − , NO 2 − and NH 4 Cl at pH 13, which are compared with those in pure 0.1 M KOH (Supplementary Fig. S27a–c ). The results indicate that the Pt-UME does not exhibit any activity for the NO 3 RR, but it can efficiently catalyze NO 2 − reduction and NH 3 oxidation in alkaline media, which is well consistent with previous studies [73] , [74] , [75] . This enables selectively detecting the in situ generated NO 2 − (at 0.06 V) and NH 3 (at 0.76 V) (Supplementary Fig. S27d–f ), when the tip of Pt-UME approaches the surface of Cu_Co(OH) 2 layer. Accordingly, a high current from NH 3 oxidation and NO 2 − reduction corresponds to a high local concentration of NH 3 and NO 2 − , respectively, above the surface of Cu_Co(OH) 2 catalyst. The SECM array scans (Fig. 3f, g ) reveal that the amount of generated NH 3 is substantially increasing at the border (X ≈ 600 μm) between the Cu and Co(OH) 2 layers, accompanying by a sharply decreased amount of generated NO 2 − . The SECM results unequivocally confirmed that the NO 2 − is preferentially formed on the Cu layer and then diffuses to the near Co(OH) 2 layer, where the NO 2 − is reduced into NH 3 according to a typical tandem catalysis process. Note that the formed NH 3 at the border of the Cu_Co(OH) 2 layers diffuses to both sides, leading to the formation of a concentration gradient around the border during the course of the SECM measurement. Identification of the active phases for NO 3 RR Ex situ XPS and Raman spectra were obtained to identify the surface phase compositions of the three catalysts (Fig. 4 , Supplementary Fig. S28 and Fig. S29 ). We find that the redox activation induced the transformation of the initial Cu/Co-based sulfide phases into the corresponding oxides and hydroxides (see detailed assignments of the XPS and Raman peaks in Supplementary Notes 1 and 2 ). As a result, CuSP consists of Cu 0 , CuO, Cu 2 O and Cu(OH) 2 [53] , [54] , [76] , whereas CoSP is composed of Co 2+ -dominated CoO and Co(OH) 2 , as well as Co 3+ -containing Co 3 O 4 and CoOOH [65] , [77] , [78] , [79] . As anticipated, CuCoSP exists as a combination of CuSP and CoSP in phase compositions, except for the observed suppression of Co 3+ –CoO x phases and increase of Cu(OH) 2 phases (Fig. 4a, b ), which points to the synergy interaction between Cu-based and Co-based phases in CuCoSP. O 1 s XPS spectra reveal a ~2-fold higher content of O vacancies on CuSP and CuCoSP than on CoSP (Fig. 4c and Supplementary Fig. S28c ) [80] . Together with the observed smaller Tafel slopes of CuSP and CuCoSP compared to CoSP (Supplementary Fig. S28f ), this result highlights a potential role of O vacancies in Cu-based phases for the initial adsorption and/or activation of free NO 3 − ions [50] , which is a key challenge for most of the reported NO 3 RR catalysts. Fig. 4: Surface phase compositions of CuSP, CoSP and CuCoSP catalysts. Cu LMM ( a ), Co 2 p 3/2 ( b ) and O 1 s ( c ) XPS spectra. d Ex situ Raman spectra. Full size image To derive the active phases for NO 3 RR experimentally, we used in situ Raman spectroscopy to monitor the phase evolution of the three catalysts at a series of applied potentials in 0.01 M KOH in the presence or absence of 0.01 M NO 3 − (Fig. 5 and Supplementary Fig. S30 ). NO 3 − ions exhibit a characteristic peak at ~1050 cm −1 [81] . K 2 SO 4 was added to ensure sufficient ionic conductivity and provides SO 4 2− ions as an external Raman reference with a typical signal at ~982 cm −1 [53] . Fig. 5: In situ Raman spectra of the catalysts and schematic of the tandem mechanisms of CuCoSP catalysts. In situ Raman spectra of CuSP ( a ), CoSP ( b ) and CuCoSP ( c ) at different applied potentials in electrolytes containing 0.01 M NO 3 − , 0.04 M K 2 SO 4 and 0.01 M KOH. d A proposed reaction mechanism of CuCoSP tandem catalysis of NO 3 RR at low overpotentials. In the middle of ( d ), the light blue region corresponds to the potential range for the reduction of NO 3 − to NO 2 species at the Cu/CuO x phases, resulting in the etching of catalysts, while the light pink region shows the potential range for efficient tandem reduction of NO 3 − to NH 3 . 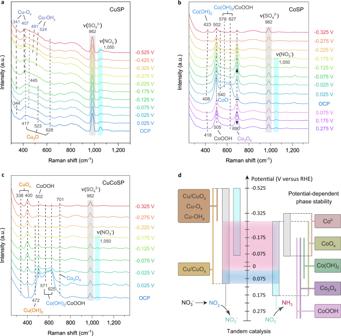Fig. 5: In situ Raman spectra of the catalysts and schematic of the tandem mechanisms of CuCoSP catalysts. In situ Raman spectra of CuSP (a), CoSP (b) and CuCoSP (c) at different applied potentials in electrolytes containing 0.01 M NO3−, 0.04 M K2SO4and 0.01 M KOH.dA proposed reaction mechanism of CuCoSP tandem catalysis of NO3RR at low overpotentials. In the middle of (d), the light blue region corresponds to the potential range for the reduction of NO3−to NO2species at the Cu/CuOxphases, resulting in the etching of catalysts, while the light pink region shows the potential range for efficient tandem reduction of NO3−to NH3. Full size image Figure 5a shows the Raman spectra of CuSP at reducing potentials related to NO 3 RR. The initial broad bands at 417, 523 and 628 cm −1 , associated with Cu 2 O phases [53] , [54] , persist at as low as −0.525 V. Remarkably, at <−0.175 V, two sets of peaks emerge at 341, 407, 491 and 524 cm −1 , previously assigned to Cu–O and Cu–OH modes, respectively [53] . The same but more notable signals are observed in the absence of NO 3 − (Supplementary Fig. S30a ), partly due to the NO 3 RR delaying the surface phase evolution. It is worth noting that CuSP can prevent poisoning only at <−0.425 V, where the surface evolution of CuSP might promote stable NH 3 generation. As a control, we further assessed the performance of a metallic Cu foil for NO 3 RR (Supplementary Fig. S14 ). The results show that at potentials >−0.425 V, Cu foil suffered from deactivation in a much higher rate, compared to CuSP containing mixed Cu/CuO x phases. Moreover, at low overpotentials, the Cu foil mainly electrochemically catalyzes the reduction of NO 3 − to highly oxidative NO 2 and acts as reducing reagents for the subsequent chemical reduction of NO 2 to NO 2 − , which is supported by the over 100% FE for NO 3 RR at −0.025 and −0.125 V (vs. RHE) (Supplementary Fig. S14c ). This chemical step will lead to the partial oxidation of metallic Cu to CuO x in alkaline electrolytes. According to recent DFT calculations on Cu and mixed Cu/Cu 2 O phase, the latter was suggested to be more active for NO 3 − to NO 2 − conversion [44] . Therefore, at low overpotentials, the catalytic nature of CuSP for NO 3 RR is related to the Cu/CuO x phases, considering the XPS-evidenced presence of Cu 0 phase. On the CoSP catalysts, the characteristic Raman peaks of multiple Co 3+ -based phases and Co(OH) 2 are fast attenuated with decreasing potentials from 0.025 V to −0.325 V (Supplementary Fig. S30b ) [77] , [78] , [79] . This indicates the gradual conversion of Co 3+ -based phases and Co(OH) 2 into CoO and metallic Co in the absence of NO 3 − [77] . In 0.01 M NO 3 − the attenuation rate of these Raman peaks was much slower (Fig. 5b ). Remarkably, the Raman signals associated with CoOOH and Co 3 O 4 phases increase at 0.025 and −0.025 V, suggesting the partial oxidation of Co 2+ in CoSP to Co 3+ [77] , [78] . Because of this, the electrolysis product of NO 3 − at 0.025 and −0.025 V should be only the highly oxidative NO 2 species in Ar-saturated alkaline electrolytes [49] , and their formation slows down the phase conversion. In this context, the Co 2+ -based phases act as chemical reducing reagents and offer additional electrons for reduction of NO 2 to NO 2 − , after which the formed NO 2 − will be electrochemically reduced to NH 3 as evidenced by the low overpotential of CoSP for the NO 2 − reduction (Fig. 3a ), finally contributing to the apparently highest FE for NH 3 at low overpotentials (Fig. 2b ). At <−0.025 V, the Raman signals of Co 3+ -based phases and Co(OH) 2 start to weaken. This result, together with the potential at −1 mA cm −2 of CoSP catalysts for NO 3 − reduction (−0.071 V), suggests that the fast reduction of NO 3 − into NO 2 − on CoSP requires the in−situ formation of metallic Co. By contrast, we found that the Co 2+ in CoSP was oxidized to Co 3+ already at >0.025 V [77] , [78] , [79] . Since the potential at −1 mA cm −2 of CoSP for NO 2 − reduction is limited to 0.176 V (Fig. 3a ), it can be concluded that the sharply increased Co 3+ -based phases at potentials >0.025 V are inactive for NO 2 − reduction. Thus, the active phase of CoSP for reducing NO 3 − to NO 2 − is related to metallic Co, while that for NO 2 − -to-NH 3 conversion is a Co 2+ -dominated CoO x phase. For CuCoSP, the Raman peaks associated with Co-based phases were quickly attenuated with decreasing potentials, while a phase assigned to CuO x emerges at 338 and 400 cm −1 (Fig. 5c and Supplementary Fig. S30c ) [54] . These results suggest an electrochemically driven phase separation in CuCoSP, leading to the formation of hybrid of Cu/CuO x and Co/CoO phases. The CuO x persists to potentials as low as −0.325 V, further decreasing the probability of in situ surface CuCo alloying, especially at potentials >−0.2 V. This is further supported by the XRD patterns, HR-TEM and EDX-mapping images of CuCoSP after repeating three electrolysis cycles of one hour at −0.325 V (Supplementary Fig. S4f and Fig. S24 ). The rate at which these Raman peaks are evolving is almost not impacted by the NO 3 RR (Fig. 5c and Supplementary Fig. S30c ). This might be attributed to the high rate of NO 3 RR on CuCoSP, which establishes a depletion layer of NO 3 − explaining the minor effects of the NO 3 RR on the phase-evolving rate. In stark contrast to CoSP (Fig. 5b ), the Raman signals of Co 3+ -based phases in CuCoSP were not enhanced at both 0.025 and −0.025 V in 0.01 M NO 3 − . This finding indicates fast reduction of NO 3 − to NO 2 − rather than to oxidative NO 2 species on the Cu-based phases of CuCoSP. Accordingly, the active Co 2+ -based phases of CuCoSP are stabilized by the Cu/CuO x phases, both of which are combined to form a tandem system for cascade NO 3 − -to-NH 3 conversion at low overpotentials (Fig. 5d ). In summary, we present a concept for designing efficient tandem catalysts, which involves the coupling of potential-dependent intermediate phases of transition metals to act as cooperative catalytic sites for cascade NO 3 − -to-NH 3 conversion. This concept was verified using Cu/CuO x –Co/CoO hybrids with a well-defined spatial arrangement that is achieved by electrochemical redox activation-induced phase reconstruction of Cu/Co-based binary metal sulfides. In this tandem catalysis system, NO 3 − ions are reduced to NO 2 − preferentially on Cu/CuO x phases, while the NO 2 − intermediates are then transferred and selectively converted to NH 3 on Co/CoO phases. The sequential NO 3 − and NO 2 − reduction on two different adjacent metal/metal oxide phases enables a high-rate NH 3 generation at low overpotentials. At −0.175 V vs. RHE, the designed CuCoSP catalysts show an excellent FE for NH 3 (90.6%) and super−high Y NH3 of 1.17 mmol cm −2 h −1 in 0.1 M NO 3 − at pH 13, outperforming most of the NO 3 RR catalysts at the same conditions. Although tandem catalysis was widely employed in heterogeneous systems, this study provides a direct demonstration of efficiently using distinct potential-dependent intermediate phases as tandem catalytic sites. This concept of splicing active phases of transition metals represents a powerful strategy towards designing high-performance, multi-functional electrocatalysts for multi-step chemical reactions, such as e.g. urea electrosynthesis by integrating NO 3 RR with CO 2 reduction. Chemicals Na 2 HPO 4 (≥99.0 %) and NaClO solution (17 %) were purchased from VWR. Maleic acid (≥99.0 %) was obtained from Riedel-de Haën. All other chemicals and Cu foil (99.98 %) were from Sigma-Aldrich. All chemicals were used without further purification. Carbon cloth was provided by PHYCHEMI. Growth of ZIF-Co-R nanorods on Cu foil and carbon cloth The Cu foil ( \(3\times 0.5\) cm 2 ) was washed with acetone, ethanol and distilled water, finally dried by blotting paper before use. The CC was initially treated with 1 M HCl (≥37%) for 12 h, washed with deionized water and dried in a 70 °C oven. Then, the CC was soaked in an aqueous solution of 2-methylimidazole (0.4 M, 99% purity) for 12 h and dried by blotting paper before use. For the growth Co-ZIF-R nanorods, the Cu foil or CC was immersed into a 14 ml growth solution, which was prepared by adding 10 ml of 2-methylimidazole (0.4 M) into 4 ml aqueous solution of Co(NO 3 ) 2 6H 2 O (50 mM, ≥98%). The Co−ZIF-R nanorods were grown under static conditions at 25 °C for 105 min. The purple Co-ZIF-R nanorods on Cu foil or CC were washed with deionized water and dried in a 70 °C oven. EC-MOF for synthesis of CuCoSP_no In a typical three-electrode system, the Co-ZIF-R on Cu foil was used as the working electrode, and Ag/AgCl (sat. KCl) and an FTO slide were employed as the reference and counter electrodes, respectively. In Ar-saturated electrolytes (aqueous solution of 0.5 M thiourea (≥99.0%), 0.25 M KCl (≥99.0%) and 0.05 M Na 2 HPO 4 ), the ZIF-Co-R was electrochemically converted via continuous CV scanning between −1.76 V and −0.15 V at a series of scan rates for different CV cycles (at 0.2 V s −1 for 1200 CV cycles, at 0.1 V s −1 for 300 CV cycles, at 0.05 V s −1 for 150 CV cycles and finally at 0.02 V s −1 for 100 CV cycles) using an Autolab potentiostat. The black products on Cu foil were taken out, rinsed with water and acetone, blow-dried by Ar gas and stored at −21 °C for further characterization. Using the same method, the CuSP_no was prepared from Cu foil directly; the CoSP_no on CC was synthesized using ZIF-Co-R nanorods on CC as precursors; the CuCoS_no on Cu foil was obtained in an electrolyte with no Na 2 HPO 4 . As a control, metallic CuCo hybrids were prepared via electrodeposition of CuCo metals and alloy on CC in 0.05 M H 2 SO 4 (98%) solution containing 4 mM CuSO 4 (≥99%) and 16 mM CoSO 4 (≥99%) at −1.75 V vs. Ag/AgCl for 400 s. Electrochemical redox activation of the samples Using a Gamry interface 1000 workstation, the samples were activated in 0.1 M KOH (≥85%) and 0.01 M potassium nitrate (≥99%) at 60 mA cm −2 for 45 s. They then underwent continuous LSV sweeping at a rate of 20 mV s −1 from −0.8 V to −1.65 V (vs. Ag/AgCl) until the polarization curves reached a steady state. This activation process was repeated two or three times. Then, the samples were gently washed with water and acetone, and dried under Ar flow for further tests or characterizations. After the redox activation, the samples of CuCoSP_no, CuSP_no, CoSP_no and CuCoS_no were named as CuCoSP, CuSP, CoSP and CuCoS, respectively. Material characterization SEM was performed using a Quanta 3D FEG scanning electron microscope. TEM images, high-angle annular dark-field TEM images, SAED patterns, element mappings and EDX line-scan were carried out on a JEOL-2800 TEM/STEM system using gold grids. XPS was recorded using an AXIS Nova spectrometer (Kratos Analytical) equipped with a monochromatic Al K α X-ray source (1487 eV, 15 mA emission current) and an inert ion gas gun for depth-profiling composition analysis as a function of etching time. For the core-level spectra, the binding energies were calibrated based on the C 1 s feature located at 284.8 eV. The nuclear magnetic resonance (NMR) spectroscopy was performed on a Bruker 400 MHz NMR spectrometer. XRD were obtained using a Bruker D8 Discover X-ray diffractometer with Cu Kα radiation ( \(\lambda =1.5418{\AA }\) ). Electrochemical NO 3 RR tests The electrochemical tests were performed using a three-electrode system connected to the Gamry workstation in a typical H-type cell. The H-type cell was separated by a Nafion 117 membrane (Dupont) that was pretreated following reported procedures [82] . The catalysts were used as the working electrode, while Ag/AgCl (3 M KCl) and platinum mesh were used as the reference and counter electrodes, respectively. The electrolytes were Ar-saturated 0.1 M KOH (pH 13) containing different concentrations of NO 3 − . The electrochemical cell was maintained in an Ar atmosphere during experiments. The LSV curves were collected at a scan rate of 5 mV s −1 . All potentials were calibrated to the RHE reference scale using \({E}_{{{{{{\rm{RHE}}}}}}}={E}_{{{{{{\rm{Ag}}}}}}/{{{{{\rm{AgCl}}}}}}}+0.207{{{{{\rm{V}}}}}}+0.0591\times {{{{{\rm{pH}}}}}}\) . The current density was normalized to the geometric electrode area (~0.5 cm 2 ). Note that the electrode area was 0.2 cm 2 for tests in 0.05 and 0.1 M nitrate. The solution resistance ( R S ) was measured using potentiostatic electrochemical impedance spectroscopy with a frequency range of 0.1 Hz to 200 kHz and an amplitude of 10 mV pp . The potentials were compensated by iR S -drop from the electrolyte resistance. Potentiostatic measurements were performed for 1 h in 30 ml cathode electrolyte with a stirring rate of 300 rpm, and then the electrolyte was stored at 4 °C (no more than 2 days) before analysis. To assess the performance change of CuCoSP during ten cycles of one-hour electrolysis at −0.175 V (vs. RHE), the electrolyte (30 ml, 0.1 M KOH and 0.01 M nitrate) was collected after each one-hour electrolysis for product analysis and a fresh electrolyte was used for the next cycle of one-hour electrolysis. Note that NH 3 volatilization in the electrolytes (pH 13) is negligible during the one-hour electrolysis (Supplementary Fig. S19 ). The C dl was determined by CV scanning in a non-faradaic potential window at different scan rates (10–120 mV s −1 ). The plot of capacitive anode and cathode current differences \([({j}_{{{{{{\rm{a}}}}}}}-{j}_{{{{{{\rm{c}}}}}}})/2]\) at a set potential against the CV scan rates shows a linear relationship, and the slope is C dl . Kinetic evaluation The LSVs of the catalysts were recorded at a scan rate of 1 mV s −1 in 0.1 M KOH (pH 13) containing 0.01 M NO 3 − or 0.01 M NO 2 − (KNO 2 , ≥96%). To obtain the rate constant, the electrolysis at −0.175 V (vs. RHE) were performed for 1 h in 22 ml electrolyte (0.1 M KOH) containing 0.01 M NO 3 − or 0.01 M NO 2 − in the cathode chamber. The reaction constant (k 1 for NO 3 − reduction and k 2 for NO 2 − reduction) was obtained by monitoring the concentration evolution of NO 3 − or NO 2 − ions as a function of electrolysis time, assuming that their concentrations decayed exponentially as per first-order rate, that is, \({C}_{{{{{{\rm{t}}}}}}}={C}_{0}{\exp }(-k\times t)\) , where, C 0 is the initial molar concentration of reactant (NO 3 − or NO 2 − ) and C t is the molar concentration of reactant at time t . Determination of ion concentrations NH 4 + quantification The produced NH 3 was quantitatively determined using the indophenol blue method [10] , [69] . Typically, a certain amount of electrolyte was taken out from the reaction cell and diluted to 2 ml. Then, 2 ml of 1 M NaOH (≥98%) solution containing sodium citrate (≥99%) and salicylic acid (≥99%) (stored at 4 °C) and 1 ml of freshly prepared 0.05 M NaClO was added. The mixed solution was shaken for few seconds. Finally, 0.2 ml of 1 wt.% sodium nitroferricyanide (≥99%) solution (stored at 4 °C) were added for the colour reaction. After keeping at room temperature for 1 h, the resulting solution was measured using an ultraviolet–visible (UV–Vis) spectrophotometer. The absorbance at ~655 nm was used to determine the concentration of NH 3 . In order to quantify the amount of NH 3 , a calibration curve was built using standard NH 4 Cl (≥99.5%) solution in 0.1 M KOH. NO 2 − quantification [44] A specific colour reagent for NO 2 − quantification was prepared by mixing 0.20 g of N-(1-naphthyl) ethylenediamine dihydrochloride (≥98%), 4.0 g of sulfonamide (≥99%) and 10 ml of phosphoric acid (85 wt.% in H 2 O) ( \({{{{{\rm{\rho }}}}}}=1.7{{{{{\rm{g}}}}}}/{{{{{\rm{ml}}}}}}\) ) with 50 ml of deionized water. In a typical colourimetric test, 1 ml HCl (1 M) was firstly added into the 5 ml of diluted post-electrolysis electrolytes, and then 0.1 ml of colour reagent was added and shaken to obtain a uniform solution. The UV–Vis absorbance at 540 nm was recorded after 20 min at room temperature. The amount of NO 2 − was determined using a calibration curve of NaNO 2 (≥96%) solutions. N 2 H 4 and NH 2 OH were probably produced during the electroreduction of nitrate. However, their concentrations are expected to be very low and only measurable at intermediate times, owing to their high reactivity in basic media [42] , [43] . Thus, we mainly focused on analyzing the yields of NH 3 and NO 2 − . NO 3 − quantification [44] , [83] A certain amount of post-electrolysis electrolytes was diluted to 4 ml. Then, 1 ml of 1 M HCl and 0.1 ml sulfamic acid (98%) solution (0.8 wt.%) were added, and the final mixed solution was shaken to obtain a uniform solution. UV–Vis spectrophotometer was used to record the absorption intensities at wavelengths of 220 nm and 275 nm. The calculated absorbance value A ( \(A={A}_{220{{{{{\rm{nm}}}}}}}-2\times {A}_{275{{{{{\rm{nm}}}}}}}\) ) is linearly related to the NO 3 − concentrations. In order to quantify the amount of NO 3 − , a calibration curve was obtained using KNO 3 standard solution. Calculation of the FE, Y NH3 and j NH3 The FE was defined as the charge consumed for the formation of a specific product (e.g., NH 3 ) divided by the total charge passing through the electrodes (Q) during electrolysis. Given that eight electrons are consumed to produce one NH 3 molecule, the FE of NH 3 (FE NH3 ), Y NH3 and j NH3 can be calculated as follows: \({{{{{{\rm{FE}}}}}}}_{{{{{{\rm{NH}}}}}}3}=(8\times {{{{{\rm{F}}}}}}\times {C}_{{{{{{\rm{NH}}}}}}3}\times V)/Q\) , \({{{{{{\rm{Y}}}}}}}_{{{{{{\rm{NH}}}}}}3}=({C}_{{{{{{\rm{NH}}}}}}3}\times V)/(A\times t)\) , and \({j}_{{{{{{\rm{NH}}}}}}3}=(Q\times {{FE}}_{{{{{{\rm{NH}}}}}}3})/(A\times t)\) , where F is the Faraday constant, C NH3 is the molar concentration of detected NH 3 , V is the volume of the electrolytes, A is the electrode geometric area, and t is the reaction time. Given that two electrons are consumed to produce one NO 2 − molecule, the FE of NO 2 − can be calculated as follows: \(\,{{{{{\rm{FE}}}}}}({{{{{{\rm{NO}}}}}}}_{2}^{-})=(2\times {{{{{\rm{F}}}}}}\times C({{{{{{\rm{NO}}}}}}}_{2}^{-})\times V)/Q\) , where C (NO 2 − ) is the molar concentration of detected NO 2 − . 15 NO 3 − Isotope labelling experiments and 14 NH 3 quantification by 1 H NMR To quantify the 14 NH 4 + yield after electrolysis of 0.01 M K 14 NO 3 at −0.175 V (vs. RHE) for 1 h, a calibration curve of 1 H NMR (400 MHz) measurements was constructed using a series of 14 NH 4 Cl solutions with defined concentrations (1, 2, 3, 4 and 5 mM) as standards. In a typical procedure [84] , 125 μl of the standard solution/electrolytes was mixed with 125 μl of 15 mM maleic acid in DMSO-D 6 (99.9 atom% D), 50 μl of 4 M H 2 SO 4 in DMSO-D 6 and 750 μl of DMSO-D 6 . The peak area integral ratio of 14 NH 4 + to maleic acid is positively correlated with the concentrations of 14 NH 4 + . To confirm the source of NH 3 qualitatively, 0.01 M Na 15 NO 3 (>98 atom% 15 N, ≥99% purity) and 0.1 M KOH were used as the feeding electrolytes for 1 h electrolysis at −0.175 V (vs. RHE) and 15 NH 4 + in the electrolyte was detected using 1 H NMR [84] . Operando SECM test To prepare the model catalyst, a CuSP slid ( \(0.5\times 3\) cm 2 ) was cleaned using 0.1 M HCl under ultrasonication for 20 min, washed by deionized water, and dried by blotting paper. Then, half of the CuSP slid was immersed in a MOFs growth solution (a mixture of 1.5 ml of 2-methylimidazole (0.4 M) and 1.5 ml aqueous solution of Co(NO 3 ) 2 6H 2 O (50 mM)) in Ar-atmosphere for 6 h. The formed Cu_ZIF-Co hybrid layers were washed with deionized water, dried with blotting paper, and further immersed in 1 M KOH solution bubbled with Ar gas for 1.5 h in a gas-tight cell, during which the ZIF-Co film was completely converted into a uniform and compacted Co(OH) 2 layer, due to the poor stability of ZIF-Co MOFs in water [85] . After washed with water and ethanol and drying at 25 °C, half of the CuSP slide was exposed in Air and the other half was covered by Co(OH) 2 nanosheets, both of which constitute the Cu (CuO x )_Co(OH) 2 model catalyst. The SECM setup with shear-force-based distance control is located in a faraday cage to allow for shielding of electrical noise, with the exception of the lock-in amplifier and the potentiostat [86] , [87] . During the SECM measurements, the Cu_Co(OH) 2 catalyst were used as the sample (working electrode 1; WE 1), while a Pt-UME with a diameter of ~1 μm (working electrode 2; WE 2), Ag/AgCl/3 M KCl (reference electrode) and a Pt-mesh (counter electrode separated by a Zirfon membrane) were assembled to a four-electrode system. The sample was polarized to −0.12 V (vs. RHE) for triggering the NO 3 RR, while at the Pt-UME cyclic voltammograms were performed in a potential range between −0.12 V and 1.58 V (vs. RHE) at a scan rate of 200 mV s −1 to identify intermediately formed NO 2 − (at 0.06 V vs. RHE) and NH 3 (at 0.76 V vs. RHE). Each SECM array scan was recorded from the Cu/CuO x layer to the Co(OH) 2 layer with an overall x-displacement of 1200 μm, while the border between the two layers is at ~600 μm. In situ Raman spectroscopy Raman spectroscopy was performed with a Lab−RAM HR Raman microscopy system (Horiba Jobin Yvon, HR550) equipped with a 532 nm laser as the excitation source, a water immersion objective (Olympus LUMFL, 60×, numerical aperture = 1.10), a monochromator (1800 grooves/mm grating) and a Synapse CCD detector. Each spectrum is an average of five continuously acquired spectra with a collection time of 50 s each. A three-electrode electrochemical cell was used for in situ Raman tests. Pt wires and Ag/AgCl (3 M KCl) were used as counter and reference electrodes, respectively. To protect the objective from the corrosive 0.1 M KOH electrolyte, 0.01 M KOH (pH 12) was used instead. K 2 SO 4 ( ≥ 99.0%) was added to ensure sufficient ionic conductivity (keeping the total concentration of K + to be 0.1 M) and provides SO 4 2− ions as an external Raman reference. Typically, in the presence of 0.01 M KNO 3 , the supporting electrolytes were 0.01 M KOH and 0.04 M K 2 SO 4 . In the absence of KNO 3 , the electrolytes were 0.01 M KOH and 0.045 M K 2 SO 4 .